A prominent and conserved role for YY1 inXisttranscriptional activation Accumulation of the noncoding RNA Xist on one X chromosome in female cells is a hallmark of X-chromosome inactivation (XCI) in eutherians. Here we uncover an essential function for the ubiquitous autosomal transcription factor Yin-Yang 1 (YY1) in the transcriptional activation of Xist in both human and mouse. We show that loss of YY1 prevents Xist upregulation during the initiation and maintenance of X-inactivation, and that YY1 binds directly the Xist 5′ region to trigger the activity of the Xist promoter. Binding of YY1 to the Xist 5′ region before XCI competes with the Xist repressor REX1, whereas DNA methylation controls mono-allelic fixation of YY1 to Xist at the onset of XCI. YY1 is thus the first autosomal activating factor involved in a fundamental and conserved pathway of Xist regulation that ensures the asymmetric transcriptional upregulation of the master regulator of XCI. X-chromosome inactivation (XCI) is a tightly regulated mechanism by which female placental mammals transcriptionally silence one X chromosome [1] . This process occurs early during development and compensate for X-linked gene dosage imbalance between males (XY) and females (XX). In most cases, XCI is random and affects either the maternal or the paternal X chromosome. Initiation of XCI strictly relies on the monoallelic upregulation of the long noncoding RNA Xist from the future inactive X (Xi) chromosome [2] , [3] , [4] . Xist transcripts accumulate on the X in cis , causing chromosome-wide transcriptional silencing and heterochromatinization [5] . One of the main challenges for dissecting early events of the random XCI process is the identification of the molecular processes and actors underlying the female-specific monoallelic upregulation of Xist and restricting it to a precise time window of development and differentiation. Mouse female embryonic stem cells (mESCs) recapitulate random XCI upon their differentiation and thus represent an adequate model system to identify XCI actors. In undifferentiated pluripotent stem cells, the Xist gene is mostly repressed; upon differentiation, the accumulation of Xist RNA that triggers X-inactivation mainly results from transcriptional activation [6] , [7] , although post-transcriptional events may also be involved [8] . Several activating and repressing factors controlling Xist expression have been described, and are for the most part encoded within an X-linked domain, encompassing Xist , known as the X-Inactivation Center ( Xic ) [9] , [10] . In addition to Xist , the Xic produces numerous noncoding RNAs, which participate to the regulation of Xist . The noncoding antisense transcript Tsix negatively regulates Xist in cis [11] ; this antisense pair of genes displays allelic mutually exclusive expression patterns at the onset of XCI. Tsix is indeed expressed from both active X chromosomes in pluripotent cells, however, upon differentiation, it is first downregulated on the future inactive X, whereas its expression is transiently maintained on the Xa [12] . Tsix has been shown to block Xist accumulation in cis during differentiation [13] , and to exert its repressive action through chromatin remodelling activities [6] , [14] , targeting in particular the Xist promoter region [15] , [16] . The noncoding RNA Jpx in contrast is required for proper Xist activation [17] and Ftx may also participate in this process [18] . The Xic also encodes RNF12, a E3-ubiquitin ligase, which acts as a dose-dependent activator of Xist [19] . RNF12, which is present in low amount in mESC, was proposed to exert its activating effect on Xist by targeting the pluripotency factor REX1 to degradation. In this model, REX1 represses Xist in mESC directly by binding to its promoter region [20] . REX1 also acts on Tsix to facilitate its transcriptional elongation [21] , [22] . During differentiation, RNF12 concentration in the nucleus increases, thus enhancing REX1 degradation rate. This would favour Xist expression and contribute to the silencing of Tsix . Tight coupling between pluripotency and Xist repression is reinforced by the action of additional core pluripotency factors such as Oct3/4 and Nanog at Xist itself [23] , Tsix [24] and Rnf12 (ref. 25 ). Although several pathways ensuring Xist repression have been described, much less is known regarding the actors that directly trigger robust Xist transcriptional activation at the onset of XCI. In addition, the extent to which Xist regulatory pathways are conserved across species is poorly addressed. Recent evidences revealed that diverse strategies have evolved in mammals to achieve XCI [26] , and these differences may rely in part on alternative modes of Xist regulation. However, robust monoallelic expression of Xist is a hallmark of XCI in all eutherians studied so far and some mechanisms for Xist activation are likely to be shared between species. We tackled the question of conserved pathways of Xist regulation using multi-species in silico analysis of the Xist promoter region. This underscored the presence of a cluster of Yin-Yang 1 (YY1)-binding sites, a few kilobases (kb) downstream of the Xist transcription start site (TSS) in every eutherian species analysed. YY1 is a multifunctional zinc finger protein that can either activate or repress transcription in a context-dependent manner. Its binding to DNA can be sensitive to DNA methylation and YY1 has been shown to bind to promoter regions of Xist [27] and Tsix [21] , [28] in the mouse. Interestingly, YY1 is phylogenetically related to REX1 as Rex1 evolved from retroposition of Yy1 ; the core binding motifs of these two proteins share some similarities [29] . Here we show that, in post-inactivation cells, YY1 binds to the Xist 5′ region in a manner that correlates with Xist expression both in mouse and in human and we identify DNA methylation as a mechanism contributing to control the mono-allelic fixation of YY1. We demonstrate that YY1 is essential for the transcriptional activation of Xist during the initiation and maintenance of X-inactivation and acts through direct activation of the Xist promoter. We, moreover, highlight a competition between YY1 and REX1 binding at the Xist 5′ region. We propose that this region acts as a platform, providing a molecular switch for the control of Xist expression. YY1 is the first autosomal activating factor involved in a fundamental and conserved pathway of Xist regulation, which ensures the asymmetric transcriptional upregulation of the master regulator of XCI. Conserved binding of YY1 to active Xist promoter in eutherian To identify conserved factors controlling Xist expression, we performed in silico analysis of Xist promoter regions in seven species of eutherian mammals ( Fig. 1a ). This analysis reveals clustered YY1 consensus binding sites in all species tested (ranging from three sites in the mouse to seven sites in dog and horse, and eight sites in humans) less than 2 kb downstream of the Xist promoter. CCCTC binding factor (CTCF)-binding sites are found in the vicinity of this cluster in rodents, but not in other branches. CTCF has been found connected to the X-inactivation process in the mouse [15] , [22] , [30] , [31] , [32] , [33] , [34] , [35] . In addition, CTCF interacts with the Cohesin complex [36] , [37] to organize chromosomal architecture [38] , [39] and RAD21 (a sub-unit of this complex) sites are also predicted in the Xist 5′ region. The most conserved pattern concerns a CTCF/RAD21 site located few kb upstream of Xist TSS in all species but rabbit. 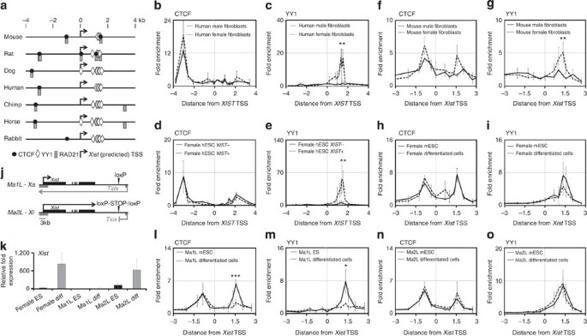Figure 1:YY1 and CTCF specifically bind the activeXistallele in human and mouse cells. (a) Map ofXist5′ region for seven eutherian species with the position of consensus binding sequences for CTCF: CC(A/G/T)(G/C)(C/T)AG(A/G)(G/T)G(A/G/T)(A/C/T)(A/G) (black dots), RAD21: CC(A/T)(G/C)(C/T)(A/G/T)G(A/G)(G/T)G(G/T)(A/C) (grey rectangles) and YY1: CGCCAT(A/T/G/C)TT (white diamonds) indicated, (b–e) ChIP analyses of CTCF and YY1 binding in human fibroblasts (IMR-90 for female, MRC-5 for male) and in female H9 hESCs expressingXIST(XIST+) or not (XIST−). Values are plotted as average fold enrichment relative to background enrichment levels. (f–i) ChIP analysis of CTCF and YY1 binding on theXistproximal region in mouse embryonic fibroblasts (MEFs), in female mESC (LF2) and in LF2 cells differentiated for 4 days using retinoic acid (RA). (j) Schematic representation ofXist/Tsixlocus in the Ma1L and Ma2L cells, with the transcriptional STOP signal truncatingTsixin Ma2L cells indicated. (k) qRT-PCR analysis ofXistexpression in female, Ma1L (male control) and Ma2L (Tsix-truncated) mESCs and their differentiated derivatives.Xistlevels are represented as fold enrichment relative to female mESCs. All samples were normalized toRplp0transcript levels. (l–o) ChIP analysis in Ma1L, Ma2L mESC and differentiated cells show maintenance of YY1 and CTCF binding specifically inXist-expressing Ma2L differentiated cells. For each panel, the average percentage of immunoprecipitation calculated for each position is plotted against the genomic location with respect to theXisttranscriptional start site (TSS, vertical line). At least three independent ChIP experiments from different chromatin extracts were carried out for each cell type. For each panel, statistical evaluation of differences is provided for the position displaying the highest enrichment; ***P<0.001; **P<0.01; *P<0.05 (Student’st-test). Error bars represent s.d. Figure 1: YY1 and CTCF specifically bind the active Xist allele in human and mouse cells. ( a ) Map of Xist 5′ region for seven eutherian species with the position of consensus binding sequences for CTCF: CC(A/G/T)(G/C)(C/T)AG(A/G)(G/T)G(A/G/T)(A/C/T)(A/G) (black dots), RAD21: CC(A/T)(G/C)(C/T)(A/G/T)G(A/G)(G/T)G(G/T)(A/C) (grey rectangles) and YY1: CGCCAT(A/T/G/C)TT (white diamonds) indicated, ( b – e ) ChIP analyses of CTCF and YY1 binding in human fibroblasts (IMR-90 for female, MRC-5 for male) and in female H9 hESCs expressing XIST ( XIST + ) or not ( XIST − ). Values are plotted as average fold enrichment relative to background enrichment levels. ( f – i ) ChIP analysis of CTCF and YY1 binding on the Xist proximal region in mouse embryonic fibroblasts (MEFs), in female mESC (LF2) and in LF2 cells differentiated for 4 days using retinoic acid (RA). ( j ) Schematic representation of Xist/Tsix locus in the Ma1L and Ma2L cells, with the transcriptional STOP signal truncating Tsix in Ma2L cells indicated. ( k ) qRT-PCR analysis of Xist expression in female, Ma1L (male control) and Ma2L ( Tsix -truncated) mESCs and their differentiated derivatives. Xist levels are represented as fold enrichment relative to female mESCs. All samples were normalized to Rplp0 transcript levels. ( l – o ) ChIP analysis in Ma1L, Ma2L mESC and differentiated cells show maintenance of YY1 and CTCF binding specifically in Xist -expressing Ma2L differentiated cells. For each panel, the average percentage of immunoprecipitation calculated for each position is plotted against the genomic location with respect to the Xist transcriptional start site (TSS, vertical line). At least three independent ChIP experiments from different chromatin extracts were carried out for each cell type. For each panel, statistical evaluation of differences is provided for the position displaying the highest enrichment; *** P <0.001; ** P <0.01; * P <0.05 (Student’s t -test). Error bars represent s.d. Full size image We used chromatin Immunoprecipitation assay (ChIP) analysis in fibroblasts and ES cells to validate these predictions and address the contribution of these binding sites to the regulation of Xist in two distantly related species, human and mouse. CTCF and RAD21 fixation upstream of Xist TSS are detected in both species ubiquitously, with no consistent difference between cells expressing Xist or not, suggesting that these bindings are not involved in controlling the asymmetric expression of Xist ( Fig. 1b,d,f,h ; Supplementary Fig. 1b,c,f,g ). This, however, does not exclude a role for these sites in other aspects of XCI. The binding of CTCF downstream of Xist TSS does correlate with Xist expression in the mouse in post-inactivation cells; it is specific to female cells, and therefore likely concerns the inactive X chromosome. However, as predicted by in silico analysis, significant binding at this position is not detected in human, at least in fibroblasts. In contrast, YY1 binding correlates with Xist expression in human and mouse contexts ( Fig. 1c,e,g,i ). It is detected in female fibroblasts but not in males in both species ( Fig. 1c,e ). In addition, in human ES cells (hESCs), YY1 is found associated with the XIST promoter region only in XIST -expressing cells. XIST indeed displays variable expression pattern in hESCs. Unlike their murine counterpart, most female hESCs have undergone XCI; XIST is initially expressed in those cells but tends to be spontaneously repressed after XCI has been established [40] . YY1 binding to the XIST 5′ region is detected in female XIST + but not in XIST − , nor in male hESCs ( Fig. 1e ; Supplementary Fig. 1e ). The binding of YY1 to Xist promoter region therefore correlates with Xist transcriptional activity in human and mouse post-inactivation cells. To explore the link between YY1 binding and Xist expression at the onset of XCI, we analysed mESCs and their differentiating derivatives. We took advantage of mutant male mESC, Ma2L, which offer the opportunity to distinguish between active and inactive X chromosomes ( Fig. 1j ). Ma2L cells carry a transcriptional stop signal terminating Tsix transcription approximately 4 kb downstream from Tsix promoter, leading to ectopic Xist upregulation and inactivation of the single X upon differentiation [15] , [41] ( Fig. 1k ). The control Ma1L cells, in which the transcriptional stop signal has been removed, behave like wild-type (WT) male cells: repression of Xist is maintained in these cells, thus preventing XCI upon differentiation ( Fig. 1j,k ). Using this system, we could show unequivocally that the binding of YY1 at Xist , while present in both undifferentiated Ma1L and Ma2L cells, is specifically maintained on the inactive X, that is, in Ma2L, during differentiation ( Fig. 1m,o ). Binding of CTCF in this context follows that of YY1 ( Fig. 1l,n ). Similar data were obtained in another Tsix mutant male cell line in which antisense transcription is strongly reduced [42] ( Supplementary Fig. 2a–d ). These results were confirmed in differentiating female cells, with binding of YY1 being maintained during differentiation ( Fig. 1i ). Moreover, in female TS cells where X-inactivation is imprinted, YY1 binding is restricted to the paternal active Xist allele ( Supplementary Fig. 2e ) [18] . Altogether, our data correlate the allelic maintenance of YY1 binding on the inactive X with the upregulation of Xist both in female cells and in Tsix mutant male cells. Allelic binding of YY1 and CTCF is DNA methylation-dependent The YY1-binding sites are embedded within the Xist promoter CpG island ( Fig. 2a ), which is methylated on the Xa and unmethylated on the Xi in differentiated cells [43] , [44] . By combining YY1 ChIP with bisulphite treatment of the immunoprecipitated material, we demonstrate that in female fibroblasts, YY1 is bound solely to the unmethylated Xist allele ( Fig. 2b ). As a control, we show that both methylated and unmethylated Xist alleles can be recovered in ChIP experiment targeting histone H3. These results confirm the allelic binding of YY1 to the active Xist promoter and are in agreement with previous reports of DNA methylation-sensitive binding of YY1 (refs 45 , 46 , 47 ). 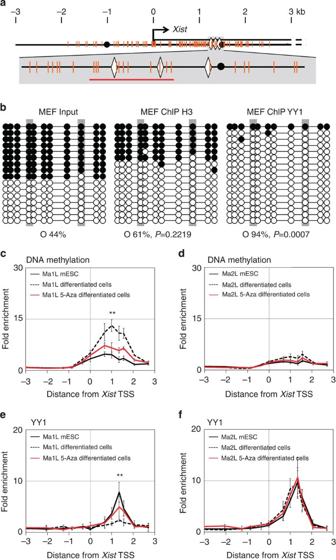Figure 2: Allelic binding of YY1 in differentiating cells is DNA-methylation dependent. (a) Top: map of the 5′ proximalXistregion as inFig. 1, with CpG dinucleotides indicated by orange vertical bars. Bottom: enlargement of the region encompassing the YY1-binding sites. (b) Bisulphite sequencing of input and DNA immunoprecipitated using the histone H3 and YY1 antibody in primary mouse embryonic fibroblasts (MEFs). Open circles and black circles represent unmethylated and methylated CpG, respectively.P-values are calculated using Fisher test comparing IP and input data. (c,d) MeDIP analysis of DNA methylation across theXistpromoter region in Ma1L and Ma2L mESC (black line), and in untreated (dotted line) and 5-aza-2′-deoxycytidine-treated (5-Aza, red line) differentiating cells. Primers amplifying regions devoid of CpG dinucleotides were used for calculating the background enrichment levels. Values are represented as fold enrichment relative to background. Three independent MeDIP experiments were performed. (e,f) ChIP analysis of YY1 binding in Ma1L and Ma2L mESCs, and in untreated and 5-Aza-treated differentiating cells. Statistical evaluation of differences between untreated and 5-aza-treated differentiated cells is provided for the position displaying the highest enrichment; ***P<0.001; **P<0.01; *P<0.05 (Student’st-test). Error bars represent s.d.,n=5. Figure 2: Allelic binding of YY1 in differentiating cells is DNA-methylation dependent. ( a ) Top: map of the 5′ proximal Xist region as in Fig. 1 , with CpG dinucleotides indicated by orange vertical bars. Bottom: enlargement of the region encompassing the YY1-binding sites. ( b ) Bisulphite sequencing of input and DNA immunoprecipitated using the histone H3 and YY1 antibody in primary mouse embryonic fibroblasts (MEFs). Open circles and black circles represent unmethylated and methylated CpG, respectively. P -values are calculated using Fisher test comparing IP and input data. ( c , d ) MeDIP analysis of DNA methylation across the Xist promoter region in Ma1L and Ma2L mESC (black line), and in untreated (dotted line) and 5-aza-2′-deoxycytidine-treated (5-Aza, red line) differentiating cells. Primers amplifying regions devoid of CpG dinucleotides were used for calculating the background enrichment levels. Values are represented as fold enrichment relative to background. Three independent MeDIP experiments were performed. ( e , f ) ChIP analysis of YY1 binding in Ma1L and Ma2L mESCs, and in untreated and 5-Aza-treated differentiating cells. Statistical evaluation of differences between untreated and 5-aza-treated differentiated cells is provided for the position displaying the highest enrichment; *** P <0.001; ** P <0.01; * P <0.05 (Student’s t -test). Error bars represent s.d., n =5. Full size image We then explored the link between DNA methylation and allelic binding of YY1 at the Xist promoter at the onset of XCI. We monitored DNA methylation in undifferentiated and differentiating Ma1L and Ma2L cells using methyl-CpG DNA immunoprecipitation (MeDIP; Fig. 2c,d ). As previously reported, the Xist CpG island is weakly methylated in undifferentiated mESC [48] and Tsix -truncated mESC cells displayed even lower methylation levels when compared with WT cells [15] . Upon differentiation, Xist DNA methylation increases by three-fold in Ma1L cells, whereas it remains low in Ma2L. These findings are reminiscent of the Xist differential methylation status observed in female somatic cells [49] . Combined with ChIP experiments performed on the same samples, our study suggests that YY1 is only bound to the unmethylated Xist CpG island, that is, in undifferentiated cells and differentiated Ma2L cells ( Fig. 2 ). To determine the functional interplay between transcription factor binding and DNA methylation, we treated differentiating Ma1L/Ma2L cells with the DNA methylation inhibitor 5-aza-2′-deoxycytidine (5-aza). As shown in Fig. 2c,d , 5-aza treatment results in drastic reduction of DNA methylation levels at the Xist CpG island in Ma1L cells, whereas it has no effect on the kinetics of differentiation as judged by the downregulation of pluripotency markers, nor on Yy1 expression levels ( Supplementary Fig. 3 ). This reduced accumulation of DNA methylation in Ma1L is accompanied by a significant maintenance of YY1 binding to Xist promoter region ( Fig. 2e , compare the red with the black dotted lines). In Ma2L cells, 5-aza treatment does not induce changes in the binding profile of YY1 ( Fig. 2f ), in agreement with DNA methylation levels being low in both untreated and treated cells. Altogether, our findings provide strong evidence that the differential DNA methylation established on the active and inactive Xist alleles at the onset of XCI controls the allelic maintenance of YY1 binding on the future inactive X chromosome. YY1 is necessary for the maintenance of Xist transcription Considering the specific binding of YY1 to the active Xist allele in human and mouse species, it is tempting to speculate that this factor contributes to the monoallelic transcription of Xist . To test this hypothesis, we performed YY1 knockdown (KD) experiments in primary human and mouse female embryonic fibroblasts, cellular contexts in which XCI is already established and Xist strongly expressed. YY1 KD in these cells reduced global YY1 RNA and protein levels ( Fig. 3a ) and abolished binding of YY1 at Xist promoter ( Fig. 3b ), but did not affect cell viability (data not shown). Notably, binding of CTCF is not affected by the loss of YY1 binding ( Fig. 3c ). YY1 KD specifically results in a strong decrease in steady-state Xist RNA levels ( Fig. 3d ) and in the number of cells displaying Xist RNA domain, as shown by RNA-fluorescence in situ hybridization (FISH) ( Fig. 3e ). These results were reproduced with two additional YY1-specific short interfering RNAs (siRNAs) targeting other regions of the YY1 transcript ( Supplementary Fig. 4 ). We then measured intronic Xist RNA levels in YY1 KD and control cells as a readout for ongoing transcription. This approach, which reveals 80% decrease in Xist premature transcript levels in the absence of YY1 ( Fig. 3f ), allows us to conclude that YY1 is essential for the maintenance of Xist transcription in mouse somatic cells. This essential role is conserved in human as XIST transcription is also severely reduced upon YY1 KD in human cells ( Fig. 3g–i ). 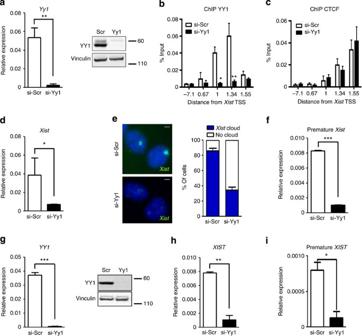Figure 3:YY1 is required for the maintenance ofXistexpression in MEFs. (a) Analysis of YY1 RNA and protein levels by qRT–PCR and western blot in female MEFs 72 h after transfection with YY1 or scramble (Scr) siRNAs. RNA expression levels are normalized toRplp0and VINCULIN is used as a loading control for protein analysis. Full western blots are presented inSupplementary Fig. 9. (b,c) ChIP analysis of YY1 and CTCF binding in si-Scr and si-YY1 KD cells. (d)Xistexpression levels as determined by qRT–PCR using primers located in contiguous exons in si-Scr and si-YY1 KD cells. (e) RepresentativeXistRNA-FISH images using the p510 probe in si-Scr and si-YY1 KD cells 72 h after transfection. Scale bars represent 5 μm. The proportion of nuclei with or withoutXistcloud is indicated (n>100). (f) Strand-specific qRT–PCR detecting intronic, prematureXistRNA levels in YY1 KD and control MEFs.Xist-specific RT primers are located in intron1 (Supplementary Table 1). Expression levels were normalized toRplp0transcript levels using gene-specific priming. (g) YY1 qRT–PCR and western blot analysis of human IMR-90 cells 72 h after transfection with YY1 or Scr siRNAs. (h,i) Quantification of spliced and prematureXISTtranscripts in the corresponding KD cells by qRT–PCR and strand-specific RT-PCR, respectively. ***P<0.001; **P<0.01; *P<0.05 (Student’st-test). Error bars represent s.d.,n=3. Figure 3: YY1 is required for the maintenance of Xist expression in MEFs. ( a ) Analysis of YY1 RNA and protein levels by qRT–PCR and western blot in female MEFs 72 h after transfection with YY1 or scramble (Scr) siRNAs. RNA expression levels are normalized to Rplp0 and VINCULIN is used as a loading control for protein analysis. Full western blots are presented in Supplementary Fig. 9 . ( b , c ) ChIP analysis of YY1 and CTCF binding in si-Scr and si-YY1 KD cells. ( d ) Xist expression levels as determined by qRT–PCR using primers located in contiguous exons in si-Scr and si-YY1 KD cells. ( e ) Representative Xist RNA-FISH images using the p510 probe in si-Scr and si-YY1 KD cells 72 h after transfection. Scale bars represent 5 μm. The proportion of nuclei with or without Xist cloud is indicated ( n >100). ( f ) Strand-specific qRT–PCR detecting intronic, premature Xist RNA levels in YY1 KD and control MEFs. Xist -specific RT primers are located in intron1 ( Supplementary Table 1 ). Expression levels were normalized to Rplp0 transcript levels using gene-specific priming. ( g ) YY1 qRT–PCR and western blot analysis of human IMR-90 cells 72 h after transfection with YY1 or Scr siRNAs. ( h , i ) Quantification of spliced and premature XIST transcripts in the corresponding KD cells by qRT–PCR and strand-specific RT-PCR, respectively. *** P <0.001; ** P <0.01; * P <0.05 (Student’s t -test). Error bars represent s.d., n =3. Full size image YY1 is necessary for Xist upregulation at the onset of XCI We next investigated the role of YY1 in the upregulation of Xist at the onset of XCI, during female ES cell differentiation. This analysis could be undertaken in mouse only. Indeed, human cells in a pre-X inactivation state are extremely rare, likely due to different kinetics of XIST expression in human pre-implantation development [26] . We developed a KD protocol in which YY1 is depleted at the undifferentiated state 2 days before the induction of differentiation, and kept at nearly undetectable levels during 4 days of differentiation ( Fig. 4a ). This ensures that YY1 is absent during the time-window of XCI initiation, both at the global level ( Fig. 4b,c ) and more specifically at the Xist 5′ region ( Supplementary Fig. 5a ). As observed in mouse embryonic fibroblasts (MEFs), CTCF remained bound to Xist in the absence of YY1 ( Supplementary Fig. 5b ). YY1 KD does not appear to affect cell differentiation, as the pluripotency factors expression profiles follow the same kinetics of downregulation in control and KD cells ( Fig. 4d ; Supplementary Fig. 5c–e ). However, YY1 KD dramatically impairs Xist upregulation, with the maximum effect observed at early stages of differentiation ( Fig. 4e ). Later on, at day 4, Xist RNA levels increase slightly but never reach the levels measured in control cells. This increase parallels the slight recovery in YY1 RNA and protein levels observed at these stages ( Fig. 4b,c ). Similar results were obtained when premature Xist RNA levels were monitored, demonstrating that, in differentiating female mESCs like in MEFs, YY1 KD affects the transcription of Xist rather than the transcript itself ( Fig. 4f ). Single-cell analysis by Xist RNA-FISH indicates that reduced Xist expression in YY1 KD cells leads to a decrease in the number of cells with a Xist RNA cloud, both at days 2 and 4 of differentiation ( Fig. 4g–i ). We thus demonstrate that YY1 is a critical factor for the appropriate upregulation of Xist and establishment of XCI during ES cell differentiation in mouse. 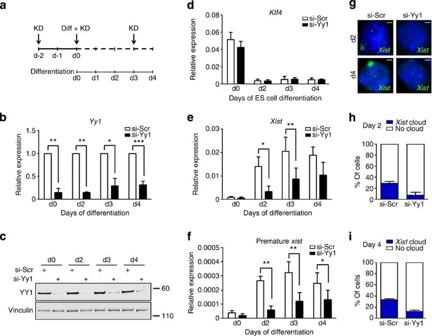Figure 4:YY1 is required for properXistupregulation at the onset of XCI. (a) Timeline indicating the YY1 KD strategy during differentiation (diff) of LF2 female mESCs. Three rounds of siRNA transfection were performed: one 2 days before the induction of differentiation (d-2), one concomitantly with the launching of differentiation (d0) and the last at day 3 (d3) of differentiation. (b) qRT-PCR and (c) western blot analysis of YY1 levels at different time points of differentiation. Expression levels are reported relative to si-Scr condition for each time point. Full western blots are presented inSupplementary Fig. 9. (d)Klf4and (e)Xistexpression levels as determined by qRT-PCR. (f) PrematureXistexpression levels determined by strand-specific qRT-PCR. (g)XistRNA-FISH on d2 or d4 of differentiation of YY1 KD and control cells. Scale bars represent 5 μm. (h–i) Quantification of nuclei (n>150) with aXistcloud at d2 (h) and d4 (i) of differentiation. ***P<0.001; **P<0.01; *P<0.05 (Student’st-test). Error bars represent s.d.,n=3. Figure 4: YY1 is required for proper Xist upregulation at the onset of XCI. ( a ) Timeline indicating the YY1 KD strategy during differentiation (diff) of LF2 female mESCs. Three rounds of siRNA transfection were performed: one 2 days before the induction of differentiation (d-2), one concomitantly with the launching of differentiation (d0) and the last at day 3 (d3) of differentiation. ( b ) qRT-PCR and ( c ) western blot analysis of YY1 levels at different time points of differentiation. Expression levels are reported relative to si-Scr condition for each time point. Full western blots are presented in Supplementary Fig. 9 . ( d ) Klf4 and ( e ) Xist expression levels as determined by qRT-PCR. ( f ) Premature Xist expression levels determined by strand-specific qRT-PCR. ( g ) Xist RNA-FISH on d2 or d4 of differentiation of YY1 KD and control cells. Scale bars represent 5 μm. ( h – i ) Quantification of nuclei ( n >150) with a Xist cloud at d2 ( h ) and d4 ( i ) of differentiation. *** P <0.001; ** P <0.01; * P <0.05 (Student’s t -test). Error bars represent s.d., n =3. Full size image YY1 competes with REX1 for binding the Xist 5′ region REX1 has been recently proposed to directly contribute to the repression of Xist in ES cells [20] . Indeed, REX1 binding to the Xist 5′ region can be detected in REX1 overexpressing cells and this is accompanied by impaired Xist accumulation upon differentiation. REX1 binding was reported to occur at two regions, one corresponding to the Xist TSS and the other overlapping the YY1-binding sites. As REX1 and YY1 consensus binding sites are highly similar [29] ( Fig. 5a ), we wanted to investigate the possibility that REX1 could compete with YY1 for binding to the Xist 5′ region. To do so, we compared REX1 and YY1 recruitment at Xist in cells with various REX1 levels. We used in particular Rex1 overexpressing and Rnf12 −/− mESCs [19] . RNF12 is an X-linked E3-ligase involved in the degradation of REX1. Xist activation and X-inactivation are impaired in differentiating Rex1 overexpressing and Rnf12 −/− cells and this was proposed to be because of the accumulation of REX1 at the Xist promoter [20] . 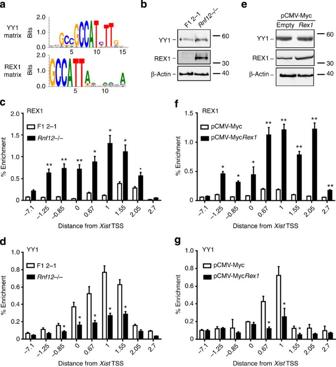Figure 5:REX1 competes with YY1 for binding to theXist5′ region. (a) REX1 and YY1 DNA binding consensus matrices. (b) Western blot analysis of YY1 and REX1 protein levels in F1 2-1 (WT) andRnf12−/−mESCs. β-Actin was used as a loading control. Full western blots are presented inSupplementary Fig. 9. (c,d) ChIP analysis of REX1 and YY1 binding in F1 2-1 WT andRnf12−/−ES cells. ChIP was performed on at least three independent chromatin extracts for each cell type. (e) Western blot analysis of YY1 and REX1 protein levels in F1 2-1 mESC transfected either with an empty pCMV-Myc (WT) or aRex1pCMV-Myc (Rex1overexpressing) vector. β-Actin was used as loading control. (f–g) ChIP analysis of REX1 and YY1 binding in control andRex1overexpressing mES cells. ChIP was performed on at least three independent chromatin extracts for each cell type. ***P<0.001; **P<0.01; *P<0.05 (Student’st-test). Error bars represent s.d. Figure 5: REX1 competes with YY1 for binding to the Xist 5′ region. ( a ) REX1 and YY1 DNA binding consensus matrices. ( b ) Western blot analysis of YY1 and REX1 protein levels in F1 2-1 (WT) and Rnf12 −/− mESCs. β-Actin was used as a loading control. Full western blots are presented in Supplementary Fig. 9 . ( c , d ) ChIP analysis of REX1 and YY1 binding in F1 2-1 WT and Rnf12 −/− ES cells. ChIP was performed on at least three independent chromatin extracts for each cell type. ( e ) Western blot analysis of YY1 and REX1 protein levels in F1 2-1 mESC transfected either with an empty pCMV-Myc (WT) or a Rex1 pCMV-Myc ( Rex1 overexpressing) vector. β-Actin was used as loading control. ( f – g ) ChIP analysis of REX1 and YY1 binding in control and Rex1 overexpressing mES cells. ChIP was performed on at least three independent chromatin extracts for each cell type. *** P <0.001; ** P <0.01; * P <0.05 (Student’s t -test). Error bars represent s.d. Full size image In WT cells, the Xist 5′ region is bound mostly by YY1. REX1 recruitment to the region is detected only in conditions in which REX1 is stabilized or overexpressed ( Fig. 5c,f ), as previously reported [20] . REX1 recruitment occurs over a broad region of the Xist 5′ end, which overlaps with and extends beyond the YY1 sites. Recruitment of REX1 in these contexts coincides with significant decrease in YY1 binding across the region ( Fig. 5d,g ). As YY1 is not a substrate for RNF12 (ref. 20 ) and YY1 levels are not affected by Rex1 overexpression ( Fig. 5b,e ), this result indicates that loss of YY1 at the Xist 5′ region is a direct consequence of REX1 occupancy of the region. Our finding thus reveals a competition between YY1 and REX1 for binding the Xist 5′ region. They also strongly suggests that the impaired upregulation of Xist in cells with elevated REX1 levels is, at least in part, due to impaired recruitment of YY1 to the region, thus confirming the importance of YY1 for Xist activation. YY1 is required for Xist promoter activity in vitro and ex vivo To confirm that YY1 directly regulates Xist expression, we tested the impact of numerous mutations of YY1-binding sites on the activity of the human and mouse Xist 5′ region in luciferase reporter assays ( Fig. 6 ). 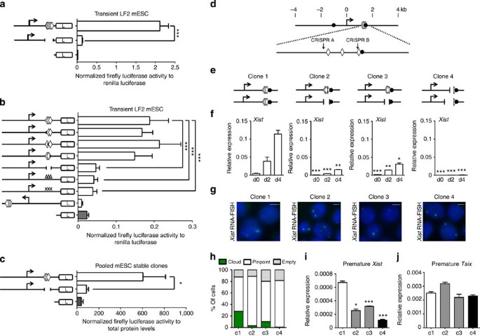Figure 6:YY1 acts onXistpromoter to controlXistactivation. (a,b) Luciferase reporter assay in female mESCs transiently transfected with WT, mutants and reverse humanXIST(a) and mouseXist(b) promoter luciferase constructs (white bars) compared with promoterless control (grey bar). White diamonds represent YY1 sites. ‘Δ’ indicate punctate deletion (10 bp) and ‘X’ point mutations of individual YY1-binding sites. Firefly Luciferase activity is reported after normalization to renilla activity, considered as internal control for transfection variability. (c) Luciferase reporter assay on pooled clones of female mESCs stably transfected with the WT luciferase construct, the construct with deletion of YY1 sites or the control promoterless vector. Normalization is performed to total protein levels. (d) Schematic view of theXist5′ region with the position of the region targeted by the two CRISPR RNAs indicated by vertical arrows. The YY1- and CTCF-binding sites are represented as diamonds and circles, respectively, and theXistTSS is indicated by a horizontal arrow. (e) Schematic view of theXist5′ region in the four clones analyzed (C1-C4), with the deletion indicated. (f) qRT–PCR analysis ofXistexpression in CRIPR/Cas9-targeted clones in ES cells (d0) and at day 2 (d2) and day 4 (d4) of a representative differentiation. Statistical evaluation of the difference between C1, considered here as WT, and clones C2–C4 carrying mutations of YY1-binding sites is provided for each day of differentiation. ***P<0.001; **P<0.01; *P<0.05 (Student’st-test). (g) RepresentativeXistRNA-FISH images of CRIPR/Cas9-targeted clones at d4 of differentiation. Scale bars represent 5 μm. (h) Quantification of nuclei (n>150) withXistRNA cloud, pinpoints or with no signal (empty) at d4 of differentiation. (i) PrematureXistexpression levels determined by strand-specific qRT–PCR at day 4 of differentiation. (j) PrematureTsixexpression levels determined by strand-specific qRT–PCR at day 4 of differentiation. Figure 6: YY1 acts on Xist promoter to control Xist activation. ( a , b ) Luciferase reporter assay in female mESCs transiently transfected with WT, mutants and reverse human XIST ( a ) and mouse Xist ( b ) promoter luciferase constructs (white bars) compared with promoterless control (grey bar). White diamonds represent YY1 sites. ‘Δ’ indicate punctate deletion (10 bp) and ‘X’ point mutations of individual YY1-binding sites. Firefly Luciferase activity is reported after normalization to renilla activity, considered as internal control for transfection variability. ( c ) Luciferase reporter assay on pooled clones of female mESCs stably transfected with the WT luciferase construct, the construct with deletion of YY1 sites or the control promoterless vector. Normalization is performed to total protein levels. ( d ) Schematic view of the Xist 5′ region with the position of the region targeted by the two CRISPR RNAs indicated by vertical arrows. The YY1- and CTCF-binding sites are represented as diamonds and circles, respectively, and the Xist TSS is indicated by a horizontal arrow. ( e ) Schematic view of the Xist 5′ region in the four clones analyzed (C1-C4), with the deletion indicated. ( f ) qRT–PCR analysis of Xist expression in CRIPR/Cas9-targeted clones in ES cells (d0) and at day 2 (d2) and day 4 (d4) of a representative differentiation. Statistical evaluation of the difference between C1, considered here as WT, and clones C2–C4 carrying mutations of YY1-binding sites is provided for each day of differentiation. *** P <0.001; ** P <0.01; * P <0.05 (Student’s t -test). ( g ) Representative Xist RNA-FISH images of CRIPR/Cas9-targeted clones at d4 of differentiation. Scale bars represent 5 μm. ( h ) Quantification of nuclei ( n >150) with Xist RNA cloud, pinpoints or with no signal (empty) at d4 of differentiation. ( i ) Premature Xist expression levels determined by strand-specific qRT–PCR at day 4 of differentiation. ( j ) Premature Tsix expression levels determined by strand-specific qRT–PCR at day 4 of differentiation. Full size image A 2.3-kb region of the human XIST promoter including the eight YY1 consensus sites confers strong activity to a luciferase reporter construct compared with an empty vector. This activity was abolished when the YY1 sites were deleted ( Fig. 6a ). Similar results were obtained with the mouse promoter region. Upon transient transfection in female mESC, the WT Xist promoter construct, which contains a 4.4-kb region encompassing the three YY1-binding sites, yields a ninefold higher luciferase activity than the corresponding promoterless vector ( Fig. 6b ). Deletion of individual YY1 and of CTCF sites does not lead to any change in the luciferase activity ( Fig. 6b ; Supplementary Fig. 6a ). In contrast, deleting a 200-bp region encompassing all YY1-binding sites significantly reduces the luciferase activity. These results, which point to an essential role for YY1 in the activity of the Xist promoter, were reproduced with smaller (10 bp) deletions or point mutations shown to block YY1 binding [27] and confirmed in stable transfectants ( Fig. 6c ). To further demonstrate the specificity of YY1 action on the Xist promoter, we knocked down YY1 in mESCs stably transfected with either mouse WT, YY1 site-deleted or promoterless luciferase constructs. Transient YY1 KD efficiently reduces YY1 RNA and protein levels in all three cell lines ( Supplementary Fig. 6b ). As shown in Supplementary Fig. 6c , YY1 KD results in a significant decrease in WT Xist promoter activity. The residual luciferase activity of the WT construct detected after YY1 KD could be due to either low remaining levels of YY1 or the implication of other factors in the activity of the Xist promoter. Nevertheless, our data demonstrate that YY1 is essential for the transcriptional activity of both the human and mouse Xist promoter in vitro . To confirm the direct contribution of YY1 to Xist regulation, we generated, in female mESC, mutations of YY1-binding sites in the Xist 5′ region using the CRISPR/Cas9 system ( Fig. 6 ; Supplementary Figs 7 and 8 ). Two guide RNAs were designed to delete the YY1-binding sites and leave the nearby CTCF site intact ( Fig. 6d ). The cutting efficiency appeared very high as most of the clones analysed displayed evidence of nicking events (data not shown). We selected four clones (C1-4) carrying two X chromosomes with various combinations of YY1-binding site sequences (WT, partially or fully deleted; Supplementary Figs 7 and 8a ). C1 carries only a partial deletion of one of the three YY1 sites on one allele, and we thus considered it as WT. In C2, one allele has lost the three YY1 sites, whereas a small deletion, which partially overlaps with the third YY1 site, is present on the other allele. C3 is mostly similar to C2, with the exception of the third site, which is only partially deleted on the two alleles. In C4, the first two YY1-binding sites have been deleted on both alleles, and the third one is also partially affected. These deletions resulted in slight (C2 and C3) or strong (C4) decrease in YY1 binding to the region, as monitored by ChIP ( Supplementary Fig. 8b ). We show that loss of YY1-binding sites impairs Xist upregulation and accumulation upon differentiation, with the most severe effects obtained in C4 ( Fig. 6f–h ; Supplementary Fig. 7c ). Decrease in Xist premature transcript levels indicate a direct, transcriptional effect of YY1 binding on Xist ( Fig. 6i ). This occurs independently of Tsix , whose expression levels are unaffected by the deletion ( Fig. 6j ). Altogether, these results indicate that YY1 binding to the Xist 5′ region has a direct and positive impact on Xist transcription. In eutherian mammals, XCI strictly depends on the mono-allelic upregulation of the noncoding transcript Xist . Once initiated in early development, robust Xist expression persists in female cells throughout development and adult life. Here, we have uncovered a major and conserved role for YY1 in the upregulation of Xist and in the maintenance of its expression. Our data strongly suggest that YY1 directly controls Xist transcriptional activation through binding to Xist 5′ region. Recently, binding of YY1 to the same cluster of sites has been proposed to tether Xist transcripts to its own locus, thus acting as a nucleation centre for Xist RNA loading on the inactive X [50] . Although our results do not exclude a role for YY1 in Xist localization, they identify an additional function for YY1 in Xist RNA metabolism. The reduced number of cells accumulating Xist RNA cloud that we observe upon YY1 KD could be interpreted as a default in Xist localization; the strong decrease in steady-state Xist RNA and pre-mature transcript levels in such cells, however, clearly indicate that YY1 activates Xist transcription, not only in the mouse but also in the human. We, moreover, provide the first targeted deletion of YY1-binding sites at the endogenous Xist locus, which allows to disentangle YY1 direct effects at Xist from more indirect ones on Xist regulators, such as Tsix (see below) and which further supports the strict requirement of YY1 for Xist upregulation. Homozygous removal of YY1-binding sites indeed resulted in a complete failure not only to accumulate Xist on the inactive X, but also to activate Xist transcription. Similar, albeit slightly reduced effects were observed in heterozygous cells. However, if YY1-binding sites served only as a nucleation centre, no difference from the WT would be expected in this context regarding both transcript levels and cloud formation, Xist upregulation would not be altered and Xist RNA would properly accumulate on the unmutated chromosome, thanks to the presence of a WT nucleation centre. In conclusion, we demonstrate using several experimental approaches, in multiple cell types and species, that preventing YY1 binding at Xist impairs Xist transcription. YY1 is, to our knowledge, the first factor shown to control Xist monoallelic expression during both initiation and maintenance phases of XCI. One exception for the stable maintenance of XCI and XIST expression is provided by female hESCs. Indeed, although most female hESCs have already undergone XCI, XIST expression was found to be highly unstable in these cells and XIST tends to be spontaneously repressed over time in culture. DNA methylation was reported to differentially mark active and repressed XIST promoters in hESCs [51] , [52] . We now provide evidence that spontaneous XIST repression in hESCs might be due to loss of YY1 binding from the XIST promoter region, likely in a DNA methylation-dependent manner. YY1 may therefore contribute to the instability of the XCI process in hESCs. YY1 also binds the Xist locus in mouse undifferentiated ES cells, which express only low levels of Xist ( Fig. 7 ). What prevents the transcriptional activating function of YY1 at the pluripotent state remains to be determined. However, it is likely that this results, at least in part, from the action of repressive mechanisms operating at this stage, in particular those mediated by Tsix and pluripotency factors binding to Xist [23] , [53] , which would overrule the transcriptional activation potentiated by YY1 binding. 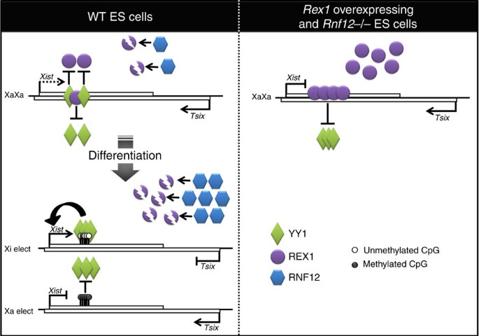Figure 7:A model recapitulating the regulation ofXistby YY1. In WT mouse ES cells, YY1 (green diamonds) binds to lowly methylatedXistallele, but this binding can be competed for by theXistrepressor REX1 (purple circles). Competition is exacerbated inRex1overexpressing and inRnf12−/−mESC, in which REX1 protein accumulates, thus leading to the displacement of YY1 fromXist. During differentiation of WT ES cells, theXistCpG island becomes asymmetrically methylated, controlling monoallelic maintenance of YY1 binding on the Xi elect. Increase in RNF12 (blue hexagons) levels enhances the degradation of REX1, reinforcing the stable binding of YY1 to the Xi, which is required forXistupregulation. Figure 7: A model recapitulating the regulation of Xist by YY1. In WT mouse ES cells, YY1 (green diamonds) binds to lowly methylated Xist allele, but this binding can be competed for by the Xist repressor REX1 (purple circles). Competition is exacerbated in Rex1 overexpressing and in Rnf12 −/− mESC, in which REX1 protein accumulates, thus leading to the displacement of YY1 from Xist . During differentiation of WT ES cells, the Xist CpG island becomes asymmetrically methylated, controlling monoallelic maintenance of YY1 binding on the Xi elect. Increase in RNF12 (blue hexagons) levels enhances the degradation of REX1, reinforcing the stable binding of YY1 to the Xi, which is required for Xist upregulation. Full size image The pluripotency factor REX1 also appears to compete with YY1 for binding at the Xist 5′ region in the mouse. Accumulation of REX1 in an Rnf12 −/− and Rex1 overexpressing contexts indeed strongly promotes YY1 displacement from Xist , which results in failure to activate Xist upon differentiation [20] . At the onset of XCI, increased concentration of RNF12 results in decreased levels of REX1, and we propose that this allows for YY1 to stably bind Xist and activate its expression ( Fig. 7 ). This activation also likely requires the action of other X-linked Xist activators such as Xpr [54] , Jpx [17] and Ftx [18] , in conjunction with the disappearance of the Xist repressive mechanisms ( Tsix and pluripotency factors). Whether the competition between REX1 and YY1 also takes place in other species remain to be investigated. YY1 is encoded by an autosomal gene and its expression, as expected, is similar in male and female cells (data not shown). Thus, YY1 female-specific action on Xist is unlikely to derive from a dose-dependent mechanism, but rather relies on allelic regulation of its binding. Our data provide evidence for the involvement of DNA methylation in the allelic maintenance of YY1 at Xist promoter on the inactive X chromosome. YY1 binding has indeed been reported as methylation sensitive, although there might be some context-dependent effects [47] , [55] . DNA methylation could therefore be sufficient for evicting YY1 and preventing the subsequent activation of Xist on the future Xa. In agreement with this, male embryos and differentiating ES cells deficient for DNA methyltransferase activity display ectopic Xist expression from their single X [56] , possibly as a result of the maintenance of YY1 binding at Xist promoter. The mechanisms underlying the establishment of differential DNA methylation at Xist have yet to be uncovered. Homologous pairing of the Xic has been recently proposed to facilitate symmetry breaking between homologous active X chromosomes and to be followed by transient Tsix mono-allelic expression [57] . Asymmetric expression of the antisense would in turn determine the X chromosomes opposite fates. Indeed, Tsix has been shown to control Xist repression in cis [11] by triggering chromatin modifications, including DNA methylation, at the Xist promoter region [7] , [15] , [16] . Interestingly YY1 also contribute to the regulation of Tsix ; YY1 binds Tsix regulatory regions and was suggested to function as a transcriptional activator for Tsix [21] , [28] . YY1 therefore appears to be a master regulatory factor for XCI, controlling the expression of Xist directly in all eutherians, and also indirectly in the mouse, through at least Tsix . As Tsix is not functionally conserved in human [58] , [59] , it will be interesting to determine whether YY1 also controls other XIST regulators in this species, but these have yet to be identified. Cell culture Mouse ES and MEF cells were grown as described previously [6] . Mouse ES cell differentiation experiments were carried out in feeder-free conditions, plated on gelatin-coated flasks at a density of 10,000 cells per cm 2 , in Dulbecco’s modified Eagle medium (DMEM), 10% fetal calf serum (GIBCO) supplemented with retinoic acid (RA) at a final concentration of 10–7 M, with the exception of differentiation of knocked down cells, for which no RA was added. Human fetal fibroblast (IMR-90 and MRC-5) cells were maintained on gelatin-coated plates in DMEM, 10% fetal calf serum medium. XIST + and XIST − human female H9 ESC lines were cultured on mitomycin C-treated MEFs in DMEM/F12 medium, supplemented with 20% of knockout serum replacement, 4 ng ml −1 β-fibroblast growth factor, 1 mM L -glutamine, 0.1 mM β-mercaptoethanol and 1% non-essential Amino Acids (GIBCO). The medium was changed daily and cells were passaged weekly with collagenase type IV (GIBCO) by scraping to obtain small clumps. Feeder cells were removed from mESC and hESC lines by adsorption before chromatin and RNA extractions. Chromatin immunoprecipitation ChIP experiments were carried out as extensively described [21] . Briefly, 20 μg of sonicated chromatin (average length 500–1,000 bp) were incubated with 2 μg of antibody overnight at 4 °C with overhead shaking. YY1 and CTCF antibodies were from Santa Cruz (sc-1703X and sc-15914X), REX1 and RAD21 from Abcam (ab50828 and ab992). Each ChIP was carried out at least three times. Real-time PCR was performed in duplicate on IP and input DNA. Primers used for ChIP analysis are provided in Supplementary Table 1 . Methylation analysis 5-Aza (Sigma) was added to the medium on day 2 of RA treatment at a final concentration of 1 μM. The medium was replaced daily until day 5 of differentiation. For the MeDIP assay, genomic DNA was sonicated to a size range of 300–1,000 bp. Ten micrograms of monoclonal antibody against 5-methylcytidine (Eurogentec, BI-MECY-0100) were used to immunoprecipitate 5 μg of denatured DNA as described in ref. 18 . Bisulphite analysis was done using previously described protocol [60] . Quantitative real-time PCR analysis Quantitative real-time PCR was performed using Power SYBR green PCR master mix in 7,500 and Viia7 Fast Real-Time PCR machines (Applied Biosystems). Primer sequences are provided in Supplementary Table 1 . To assess the enrichment of each target genomic region after MeDIP or ChIP, we calculated the ratio between the average value obtained for the IP DNA and the corresponding input, both values being first normalized for dilution factors. Results obtained were normalized to average background signal leading to fold enrichment values except in Fig. 5 where results are presented as percentage of enrichment. Reverse transcription (RT)-PCR and strand-specific RT-PCR Total RNA was extracted using Trizol reagent and treated with Turbo DNAse 20 min 37 °C (Life Technologies). RNA of 0.5–1 μg were random primed reverse-transcribed at 42 °C using Vilo reverse-transcriptase (Life technologies). Control reactions lacking enzyme were systematically run and verified negative for all samples. Expression levels were normalized to either Rplp0 (mouse cells) or GAPDH (human cells) transcript levels. Strand-specific RT-PCR was performed to detect the premature Xist transcript using primers detecting Xist (sense orientation) or Tsix (antisense orientation) together with Rplp0 -specific primer for normalization. 250 ng of DNase-treated RNA extracts were reverse transcribed with SuperScript III reverse-transcriptase at 55 °C. Control reactions lacking enzyme or primers were verified negative. Control reactions testing each primer individually were also carried out to exclude cross reaction between primers. RNA-FISH MEFs were grown on coverslips, whereas differentiating ES cells were cytospun onto SuperfrostPlus slides (VWR). Cells were permeabilized in CSK freshly supplemented with 1 mM EGTA/0.5% Triton X-100/2 mM Vanadyl Ribonucleoside Complex (Biolabs) on ice for 5 min, fixed with 1 × PBS/3% paraformaldehyde for 10 min and progressively dehydrated in ethanol. For XIST RNA detection, a 19-kb DNA probe [61] was labelled with digoxigenin using the bioprime random priming kit (Life Technologies). Hybridization was carried out overnight at 37 °C and washed three times in 50% formamide/2 × SSC at 42 °C, and three times in 2 × SSC at 42 °C. Coverslips/slides were incubated with a FITC-conjugated anti-DIG antibody (Roche, 1:250) for 20 min at 37 °C. Three additional washes with 4 × SSC/0.1% Tween-20 at 37 °C were performed and coverslips were mounted on slides in Vectashield containing DAPI and visualized under fluorescent microscope. Transient and stable transfections and luciferase assay A 4.4 kb of the mouse Xist 5′ region and either a 2.3 kb or a 1.6 kb of the human XIST 5′ region was PCR amplified, cloned into pGl4.10 [luc2] promoterless vector (Promega). The full-length mouse Xist plasmid served as a template for the generation of other single or combined deletion carrying constructs. Mutagenesis was carried out using the lightning site-directed mutagenesis kit (Agilent technologies). Primers were designed with the manufacturer’s dedicated programme (QuikChange Primer design). LF2 female ES cells were transiently transfected (Fugene transfection reagent, Promega) with human or mouse promoter constructs together with an internal control Renilla reporter vector, plGl4.74 [hRluc/TK] (Promega). Cells were lysed 48 h post transfection and Luciferase activity was measured using the Dual Luciferase reporter assay system on a GloMax multi-detection system instrument (Promega). Stable population of female LF2 ES cells were generated by co-transfection of reporter construct with a neomycin selection vector. Luciferase activity was assessed using the Bright Glo Luciferase assay system (Promega). Results were normalized to total protein amounts present in cell lysates. For REX1 overexpression studies, Rex1 cDNA was cloned in pCMV-Myc (Clontech) using primers provided in Supplementary Table 1i . Stable populations of F1 2-1 ES cells were generated by co-transfection of the pCMV-Myc empty or Rex1 -containing vector with a neomycin selection plasmid. siRNA transfection and Western analysis Control and YY1-specific siRNAs were purchased from (Sigma-Aldrich). siRNA target sequences are reported in Supplementary Table 1 . Differentiated mouse and human cells were transfected using Lipofectamine RNAi Max (Life Technologies) with a final concentration of 60 nM of siRNA. Cells were collected 72 h post transfection for RNA and protein extractions, or fixed and permeabilized for RNA-FISH procedure. For YY1 depletion during ES cell differentiation, three transfection procedures were performed at different time points (d-2, d0 and d3). KD was confirmed by RT-PCR and western blotting with αYY1 (1:500, Santa Cruz, sc-1703) and αVINCULIN (1:5,000, V9131 Sigma Aldrich). For REX1 overexpression studies, antibodies against REX1 (1:500 Abcam, ab50828) and β-ACTIN (1:5,000, A5316 Sigma Aldrich) were used. YY1 and REX1 DNA-binding matrices To determine the consensus binding sequences of YY1 and REX1, previously published ChIP-seq experiments ( GSE31785 and GSE36417 respectively) were reanalysed (mapping using bowtie1 on mm9 genome using the option: -t -q -p 8 -S -n 2 -e 70 -l 50--maxbts 125 -k 1 -m 1 (ref. 62 ). We extracted the sequences of the 250 top binding sites (HOMER peak calling, available at http://biowhat.ucsd.edu/homer/ ) and performed de novo motif discovery using MEME [63] . CRISPR/Cas9 deletion of YY1-binding sites The CRISPR/Cas Nucleases system was used to delete the YY1-binding sites in female mouse ES cells, leaving the CTCF-binding site intact. Two target regions were selected: region A positioned upstream of the first YY1-binding site and region B spanning the third site. Positioning the guide RNA target sequence on the site 3 was constrained by the presence of the CTCF site 14 bp downstream. DNA oligonucleotides harbouring the sgRNA target sequences were designed using the ZiFiT Targeter programme ( http://zifit.partners.org/ZiFiT/Disclaimer.aspx ). Oligonucleotide pairs were annealed to generate short double-stranded DNA fragments with overhangs compatible with ligation into the Bsm BI-digested plasmid pMLM3636. The Cas9 expression plasmid pJDS246 and the sgRNA expression plasmid pMLM3636 were obtained from Addgene (Addgene #43860 and #47754). How to cite this article: Makhlouf, M. et al . A prominent and conserved role for YY1 in Xist transcriptional activation. Nat. Commun. 5:4878 doi: 10.1038/ncomms5878 (2014).